Involvement of Bag6 and the TRC pathway in proteasome assembly The 26S proteasome has an elaborate structure, consisting of 33 different subunits that form the 20S core particle capped by the 19S regulatory particle on either end. Several chaperones that are dedicated to the accurate assembly of this protease complex have been identified, but the mechanisms underlying proteasome biogenesis remain unexplored so far. Here we report that core particle assembly becomes less efficient if the TRC pathway, which mediates insertion of tail-anchored proteins, is defective. We demonstrate that Bag6, a protein in the TRC pathway that is also responsible for the degradation of mislocalized proteins, is not only involved in core particle assembly but also has a key role in efficient regulatory particle assembly by directly associating with precursor regulatory particles. These findings indicate that proteasome assembly is not solely mediated by dedicated chaperones but also depends on general chaperones that preserve protein homeostasis. The 26S proteasome is an ATP-dependent protease responsible for the degradation of ubiquitinated proteins [1] . Protein degradation by the proteasome regulates diverse cellular processes including cell cycle, DNA repair, signal transduction and protein quality control by catalysing selective elimination of regulatory proteins and damaged proteins [2] . This large protein complex is composed of the catalytic 20S core particle (CP, also called the 20S proteasome) and the 19S regulatory particle (RP, also called PA700 in mammals), which is attached to either or both ends of the CP. The CP is a cylindrical-shaped stack of four heptameric rings, in which the outer rings and inner rings are each composed of seven homologous α-subunits (α1–α7) and seven homologous β-subunits (β1–β7), respectively. The proteolytic active sites reside within the central chamber enclosed by the two inner β-rings while a small channel formed by the outer α-ring, which is primarily closed, restricts the access of most native proteins to the catalytic chamber [3] . Association of the RP with the α-rings confers ubiquitin- and ATP-dependent protein degradation activity on the 26S proteasome. The RP consists of 19 different subunits and can be divided into two subcomplexes: the base and the lid [4] . The base is composed of six different homologous AAA-ATPase subunits, Rpt1–6, and three non-ATPase subunits, Rpn1, Rpn2 and Rpn13. The ATPase subunits form a hexameric ring and are required not only for substrate unfolding using energy liberated from ATP hydrolysis but also for α-ring channel opening exerted by the carboxy (C)-termini of Rpt2 and Rpt5 (refs 5 , 6 , 7 ), which are the prerequisites for threading substrates into the CP. Ubiquitinated proteins are recognized by the base subunits Rpn1 and Rpn13, either directly or indirectly. Another RP subunit Rpn10 also captures ubiquitinated proteins. The ubiquitin chains of captured substrates are cleaved by the lid. The lid is composed of nine non-ATPase subunits, Rpn3, Rpn5–9, Rpn11–12 and Rpn15 (also called Sem1 in yeast and DSS1 in mammals), in which the metalloisopeptidase Rpn11 has an essential role in deubiquitination of the substrates [8] , [9] . Recent studies using cryo-electron microscopy and single-particle analysis clarified the subunit arrangement within the 26S proteasome, which provides mechanistic insights into how the proteasome coordinates complex activities required for degradation of ubiquitinated proteins [10] , [11] , [12] . These results also indicate that accurate proteasome assembly is essential for protein degradation. However, the exact assembly mechanism of this elaborate structure consisting of the 33 different proteasome subunits is still not well understood. Considerable progress has been made recently in understanding both CP and RP assembly. CP assembly is supported by multiple proteasome-dedicated chaperones such as PAC1-4 and UMP1 (also known as POMP or Proteassemblin) in mammals, and Pba1-4 and Ump1 in yeast. These chaperones help α-ring formation and β-subunit recruitment on the α-ring, resulting in the formation of half-CPs, which then dimerize and yield active CPs, accompanied by autocatalytic processing of β-subunit propeptides and degradation of PAC1, PAC2 and UMP1 [13] , [14] , [15] , [16] . The assembly of the base subcomplex of the RP is also facilitated by specific chaperones called p28/gankyrin, p27, S5b and Rpn14 in mammals, and Nas6, Nas2, Hsm4 and Rpn14 in yeast [17] , [18] , [19] , [20] , [21] , [22] . The base subunits and these chaperones are assembled into three modules, which then associate to yield the base subcomplex. The assembly pathway of the lid subcomplex has also been demonstrated, although no chaperones seem to be involved in its assembly [23] , [24] . In this study, beginning with a genetic screen for mutants that showed synthetic growth defect with nas6Δ in yeast, we identified the involvement of the TRC/GET pathway, which mediates membrane insertion of tail-anchored (TA) proteins, in the CP assembly. We also revealed that Bag6, which is a multifunctional chaperone that has a role in the TRC/GET pathway and also in the degradation of mislocalized/misfolded proteins, is not only involved in CP assembly through the TRC/GET pathway but also in RP assembly by directly associating with precursor RPs. Our results indicate that proteasome assembly is not solely mediated by dedicated chaperones but also by chaperones that have wider roles in protein homoeostasis. Genetic interactions of Get3 with assembly chaperones In search of molecules involved in proteasome-dependent protein degradation, we employed a synthetic genetic array (SGA) analysis in Saccharomyces cerevisiae [25] using a strain lacking Nas6, an assembly chaperone for the RP [17] , [18] , [19] , [20] , [21] , as a query. This screening identified Get3, whose deletion caused synthetic growth defect with nas6Δ at high temperature ( Fig. 1a ). GET3 also showed genetic interactions with other proteasome assembly chaperones such as HSM3 , RPN14 and UMP1 (refs 17 , 18 , 19 , 20 , 21 , 22 , 26 , 27 ). These results suggest the involvement of Get3 in proteasome function ( Fig. 1b–d ). 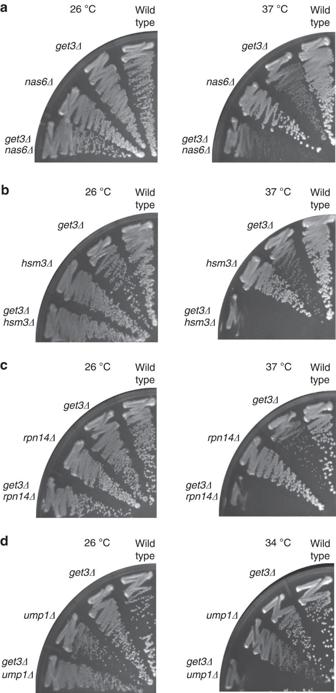Figure 1: Synthetic growth defect ofget3Δwith the deletion of proteasome assembly chaperones. (a–d) The indicated strains were streaked on YPAD and incubated at 26 °C (left panels) or at the indicated non-permissive temperature (right panels) for 2 days. Figure 1: Synthetic growth defect of get3Δ with the deletion of proteasome assembly chaperones. ( a – d ) The indicated strains were streaked on YPAD and incubated at 26 °C (left panels) or at the indicated non-permissive temperature (right panels) for 2 days. Full size image TRC40 is involved in CP assembly in mammals Get3 is a yeast orthologue of the mammalian Transmembrane Recognition Complex subunit of 40 kDa (TRC40), a central component of the TRC pathway, through which TA proteins are delivered to the endoplasmic reticulum (ER) for membrane insertion [28] , [29] . The TRC pathway (the GET pathway in yeast) comprises a ribosome-bound Bag6-TRC35-Ubl4A complex (Sgt2-Get4-Get5), cytosolic TRC40 (Get3) homodimer and an ER-localized receptor complex (unestablished in mammals; Get1-Get2 in yeast) [30] ( Supplementary Fig. S1 ). We next examined whether TRC40 is engaged in proteasome function in mammalian cells. Knockdown of TRC40 in HEK293T cells increased ubiquitinated proteins in cells ( Fig. 2a ) and reduced peptidase activity of the proteasome, especially in 20S fractions ( Fig. 2b , fractions 14–18). In addition, hallmarks of immature CPs were observed in TRC40-knockdown cells; levels of β2 and β5 subunits with propeptides and the dedicated chaperone UMP1, which are cleaved or degraded upon CP maturation [14] , were increased compared with control cells, whereas the amount of the base subunit Rpt6 and the lid subunit Rpn3 were nearly equal, suggesting a defect in CP assembly in the absence of TRC40 ( Fig. 2c ). 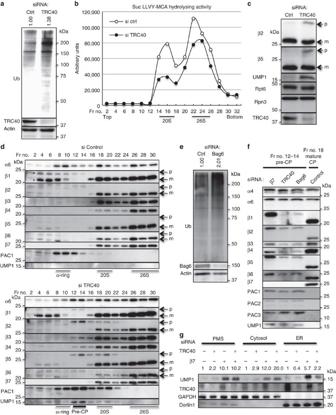Figure 2: TRC40 and Bag6 are involved in CP assembly. (a,c) Immunoblot analysis of extracts of HEK293T cells treated with siRNA targeting TRC40 or control siRNA. p, precursor; m, mature. Values for the relative band intensities of ubiquitin normalized to actin are shown ina. (b) The cell extracts inawere fractionated by 8–32% glycerol gradient centrifugation and assayed for Suc-LLVY-MCA hydrolysing activity. Representative data from five independent experiments are shown. (d) Extracts of cells treated asawere fractionated by 4–24% glycerol gradient centrifugation, and the resultant fractions were immunoblotted with the indicated antibodies. Asterisks indicate nonspecific bands. p, precursor; m, mature. (e) Immunoblot analysis of extracts of HEK293T cells treated with siRNA targeting Bag6 or control siRNA. Values represent as ina. (f) Cells were transfected with siRNAs targeting β7, TRC40 or Bag6, lysed, and fractionated by 4–24% glycerol gradient centrifugation. Fractions 12–14 that included pre-CPs were immunoblotted with the indicated antibodies. These were compared with fraction 18 of control cells (mature CPs). Approximately equimolar amounts of α-subunits were loaded. (g) Cells were transfected with siRNAs targeting β7 and TRC40 in the indicated combinations, fractionated into post-mitochondrial supernatant, cytosol and ER fractions, and subjected to immunoblot analysis. GAPDH and Derlin1 were probed as loading controls for the cytosol and the ER, respectively. Values for the relative band intensities of UMP1 normalized to GAPDH (PMS and cytosol) or Derlin1 (ER) are shown, with the control knockdown of each fraction being set to one. Figure 2: TRC40 and Bag6 are involved in CP assembly. ( a , c ) Immunoblot analysis of extracts of HEK293T cells treated with siRNA targeting TRC40 or control siRNA. p, precursor; m, mature. Values for the relative band intensities of ubiquitin normalized to actin are shown in a . ( b ) The cell extracts in a were fractionated by 8–32% glycerol gradient centrifugation and assayed for Suc-LLVY-MCA hydrolysing activity. Representative data from five independent experiments are shown. ( d ) Extracts of cells treated as a were fractionated by 4–24% glycerol gradient centrifugation, and the resultant fractions were immunoblotted with the indicated antibodies. Asterisks indicate nonspecific bands. p, precursor; m, mature. ( e ) Immunoblot analysis of extracts of HEK293T cells treated with siRNA targeting Bag6 or control siRNA. Values represent as in a . ( f ) Cells were transfected with siRNAs targeting β7, TRC40 or Bag6, lysed, and fractionated by 4–24% glycerol gradient centrifugation. Fractions 12–14 that included pre-CPs were immunoblotted with the indicated antibodies. These were compared with fraction 18 of control cells (mature CPs). Approximately equimolar amounts of α-subunits were loaded. ( g ) Cells were transfected with siRNAs targeting β7 and TRC40 in the indicated combinations, fractionated into post-mitochondrial supernatant, cytosol and ER fractions, and subjected to immunoblot analysis. GAPDH and Derlin1 were probed as loading controls for the cytosol and the ER, respectively. Values for the relative band intensities of UMP1 normalized to GAPDH (PMS and cytosol) or Derlin1 (ER) are shown, with the control knockdown of each fraction being set to one. Full size image The CP comprises 28 subunits arranged in a cylindrical particle containing four heteroheptameric rings: αββα [1] . The assembly of the mammalian CP starts with the formation of the α-rings composed of α1–α7 assisted by dedicated assembly chaperone complexes PAC1-PAC2 and PAC3-PAC4. β-subunits are then recruited onto the α-ring with the help of UMP1, except for β7, in the order β2, β3, β4, β5, β6 and β1, some of which are in immature forms with propeptides, resulting in half-CP complexes. Half-CPs then dimerize on the incorporation of β7 to form mature CPs, accompanied by cleavage of β-subunit propeptides and degradation of UMP1 and PAC1-PAC2 ( Supplementary Fig. S1 ) [14] , [26] , [31] , [32] , [33] , [34] , [35] , [36] . To better resolve the assembly defect in TRC40-knockdown cells, cell lysates fractionated using glycerol gradient centrifugation were subjected to immunoblotting ( Fig. 2d ). A notable finding was that precursor forms of CPs (pre-CPs) composed of α-rings and precursor β-subunits, as well as assembly chaperones PAC1 and UMP1, were accumulated in the absence of TRC40 ( Fig. 2d , fractions 12–14). Precursor β-subunits, PAC1 and UMP1, which should be processed or degraded before the completion of CP assembly, were observed even at 20S fractions of the knockdown cells ( Fig. 2d , fractions 18–20). These results demonstrate that TRC40 is required for efficient CP assembly, in particular in the process of productive dimerization of half-CPs. The whole TRC pathway is involved in CP assembly To examine whether not only TRC40 but also other components of the TRC pathway are involved in CP assembly, we employed the knockdown of Bag6 (also known as Bat3 or Scythe), which is the most upstream component of the TRC pathway that together with TRC35 and Ubl4A captures TA proteins at the ribosome and loads them onto TRC40 [37] , [38] . Bag6-knockdown cells accumulated ubiquitinated proteins ( Fig. 2e ) and exhibited a defect in CP assembly quite similar to TRC40 knockdown with respect to the accumulation of pre-CPs in fractions 12–14 and presence of β-subunits with propeptides as well as assembly chaperones in 20S fractions ( Supplementary Fig. S2a ). These results demonstrate that defect in either TRC40 or Bag6 causes the same defect in CP assembly and suggest that the TRC pathway as a whole has an important role in efficient CP assembly. This notion was further supported by the observations that the deletion of Get1 and Get2, the most downstream components of the GET pathway (the equivalent of the mammalian TRC pathway in yeast) [30] , [39] , caused synthetic growth defect with nas6Δ , which is particularly obvious at high temperature ( Supplementary Fig. S2b ). The defective TRC pathway impairs β-subunit assembly To clarify components of the assembly intermediates observed in cells depleted of TRC40 and Bag6, these intermediates were compared with mature CPs, which should contain equal amounts of each CP subunits, and with the intermediates that were produced by β7 knockdown and thus should contain assembly chaperones UMP1 and PAC1-PAC2 and CP subunits, except β7 (refs 34 , 35 , 36 ) ( Fig. 2f ). When the samples were loaded so as to provide comparable amounts of α4 and α6, it turned out that intermediates in both TRC40- and Bag6-knockdown cells contained UMP1 and PAC1-PAC2 as well as all the β-subunits, except β7, of which β1, β2, β5 and β6 were in unprocessed proforms, similar to the ones seen in β7-knockdown cells. However, much fewer β-subunits were present in the intermediates of TRC40- and Bag6-knockdown cells compared with mature CPs and the intermediates of β7-knockdown cells, indicating inefficient β-subunit assembly on α-rings in the absence of TRC40 and Bag6 ( Fig. 2f ). Another difference is the increased level of PAC3 in the intermediates of TRC40- and Bag6-knockdown cells compared with β7-knockdown cells ( Fig. 2f ). PAC3 is associated with α-rings and detaches from them on β3 recruitment [36] . A small amount of PAC3 was already observed in the intermediates by β7 knockdown, which in principle halts the CP assembly just before β7 incorporation, suggesting that such intermediates are unstable and that some of the already incorporated β-subunits detach. This view is supported by the observation that some of the β-subunits, especially β3, β4 and β6, but not β5, were markedly decreased in β7-knockdown intermediates compared with those in mature CPs ( Fig. 2f ). In TRC40- and Bag6 knockdowns, more PAC3 and less β-subunits were included in the intermediates, compared with those of β7-knockdown. This observation implies that a wide range of intermediates during β-subunits incorporation, from α-rings to half-CPs, are present in these intermediates ( Supplementary Fig. S1 ). This therefore suggests that TRC40 and Bag6 has a role in efficient β-subunit assembly on α-rings, possibly either by promoting the recruitment of β-subunit on the α-rings or by increasing the stability of CP-assembly intermediates. To understand the mechanism by which TRC40 and Bag6 are involved in CP assembly, we examined whether they physically associate with CP-assembly intermediates or CP subunits and chaperones. However, we did not detect any such interaction by either immunoprecipitation experiments or by yeast two-hybrid assay ( Supplementary Fig. S3a–d ). These results suggest that TRC40 and Bag6 are involved in CP assembly indirectly through the TRC pathway and lead to the assumption that a certain TA protein that is a substrate of the TRC pathway is potentially responsible for efficient CP assembly. It has been shown previously that pre-CPs are mainly associated with the ER membrane [40] . To test whether a defect in the TRC pathway affects ER association of pre-CPs, cell fractionation experiments were performed with cells treated with or without short interfering RNAs (siRNAs) targeting TRC40 and β7. Whereas the total amount of pre-CPs was increased in TRC40-knockdown cells compared with control cells, as shown by immunoblotting for UMP1, ER-associated pre-CP levels were somewhat decreased ( Fig. 2g ; lanes 1, 2, 9 and 10). In order to discern this effect more clearly, β7 knockdown was employed to increase the amount of pre-CPs. The amounts of total pre-CPs were comparable between TRC40/β7-double knockdown and β7-single knockdown ( Fig. 2g ; lanes 3 and 4). However, again as expected, decrease in ER-associated pre-CPs was observed while cytosolic pre-CPs increased in TRC40/β7-double knockdown cells compared with β7-single knockdown cells ( Fig. 2g ; lanes 7, 8, 11 and 12). These results indicate that a defect in the TRC pathway diminishes the association of pre-CPs with the ER membrane, which might be a major cause of inefficient CP assembly. Defect in RP assembly in Bag6-knockdown cells An intriguing feature of Bag6 knockdown is that, despite a defect in CP assembly, it increased free CPs and decreased 26S proteasomes, a pattern often observed when RP assembly is defective [17] , [18] , [19] , [20] , [21] ( Fig. 3a ). The RP can be divided into base and lid subcomplexes. The base comprises Rpt1-Rpt6, Rpn1, Rpn2 and Rpn13, and its assembly is preceded by the formation of three distinct modules named p28 (p28-Rpt3-Rpt6-Rpn14 complex), S5b (S5b-Rpt1-Rpt2-Rpn1 complex) and p27 modules (p27-Rpt4-Rpt5 complex), in which the assembly chaperones p28, Rpn14, S5b and p27 regulate the association between the modules and between the RP and CP in mammals [17] , [18] , [19] , [20] , [21] . 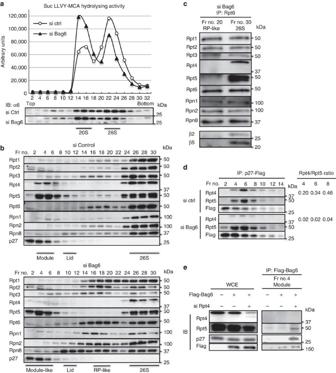Figure 3: Bag6 mediates the incorporation of Rpt4 into the p27-Rpt5 complex. (a) Cell extracts of HEK293T cells treated with siRNA-targeting Bag6 or control siRNA were separated by 8–32% glycerol gradient centrifugation and assayed for Suc-LLVY-MCA hydrolysing activity. Representative data from five independent experiments are shown. (b) Cell extracts prepared as inFig. 2ewere separated by 4–24% glycerol gradient centrifugation. The resultant fractions were immunoblotted with the indicated antibodies. Asterisks indicate nonspecific bands. (c) Fractions 20 and 30 in (b) were immunoprecipitated with the anti-Rpt6 antibody. Approximately equimolar amounts of RP subunits except Rpt4 and Rpt5 were loaded and immunoblotted with the indicated antibodies. (d) HEK293T cells stably expressing p27-Flag were treated with siRNA targeting Bag6 or control siRNA. Their cell extracts were separated by 4–24% glycerol gradient centrifugation, followed by immunoprecipitation of fractions 2–14 with an anti-Flag antibody and immunoblot analysis with the indicated antibodies. Values represent the band intensities of Rpt4 relative to those of Rpt5 in fractions 4, 6 and 8. (e) HEK293T cells stably expressing Flag-Bag6 were treated with siRNA targeting Rpt4 or control siRNA, and whole-cell extracts (WCE) were separated by 4–24% glycerol gradient centrifugation. Fraction 4 that included the p27 module or its incomplete form was immunoprecipitated with an anti-Flag antibody and immunoblotted with the indicated antibodies. Figure 3: Bag6 mediates the incorporation of Rpt4 into the p27-Rpt5 complex. ( a ) Cell extracts of HEK293T cells treated with siRNA-targeting Bag6 or control siRNA were separated by 8–32% glycerol gradient centrifugation and assayed for Suc-LLVY-MCA hydrolysing activity. Representative data from five independent experiments are shown. ( b ) Cell extracts prepared as in Fig. 2e were separated by 4–24% glycerol gradient centrifugation. The resultant fractions were immunoblotted with the indicated antibodies. Asterisks indicate nonspecific bands. ( c ) Fractions 20 and 30 in ( b ) were immunoprecipitated with the anti-Rpt6 antibody. Approximately equimolar amounts of RP subunits except Rpt4 and Rpt5 were loaded and immunoblotted with the indicated antibodies. ( d ) HEK293T cells stably expressing p27-Flag were treated with siRNA targeting Bag6 or control siRNA. Their cell extracts were separated by 4–24% glycerol gradient centrifugation, followed by immunoprecipitation of fractions 2–14 with an anti-Flag antibody and immunoblot analysis with the indicated antibodies. Values represent the band intensities of Rpt4 relative to those of Rpt5 in fractions 4, 6 and 8. ( e ) HEK293T cells stably expressing Flag-Bag6 were treated with siRNA targeting Rpt4 or control siRNA, and whole-cell extracts (WCE) were separated by 4–24% glycerol gradient centrifugation. Fraction 4 that included the p27 module or its incomplete form was immunoprecipitated with an anti-Flag antibody and immunoblotted with the indicated antibodies. Full size image We investigated the distribution of RP subunits fractionated using glycerol gradient centrifugation ( Fig. 3b ). Notably, an RP-like complex that contained RP subunits, except Rpt4 and Rpt5, was accumulated in fractions 18–20 in Bag6-knockdown cells ( Fig. 3b ). To verify the composition of this complex, fraction 20 (RP-like) and fraction 30 (26S) were immunoprecipitated with an anti-Rpt6 antibody. Immunoblot analysis showed that the RP-like complex was specifically deficient in Rpt4 and Rpt5 while containing all the other base subunits and a lid subunit ( Fig. 3c ), suggesting that RP assembly was compromised in the absence of Bag6 because of defective incorporation of Rpt4 and Rpt5. This raises the possibility that the function of the p27 module is impaired [21] . Bag6 binds to Rpt5 for assembly of the p27 module The p27 module was readily found around fraction 6 in control cells ( Fig. 3b,d ). In contrast, in Bag6-knockdown cells, Rpt4 almost completely disappeared from these fractions and Rpt5 was shifted to lighter fractions ( Fig. 3b ). In these fractions of Bag6-knockdown cells, p27 was associated with Rpt5 and Rpt4 was co-immunoprecipitated with p27 only faintly, compared with control cells ( Fig. 3d ). These results indicate that Bag6 supports the incorporation of Rpt4 into the p27-Rpt5 complex. To see whether Bag6 is associated with components of the p27 module, extracts of cells stably expressing Flag-Bag6 that were transfected with either control or Rpt4-targeting siRNA were fractionated using glycerol gradient centrifugation ( Supplementary Fig. S4 ). In control cells, the p27 module was found in fractions 4–6, whereas Rpt5 and p27, but not Rpt4, were observed in these fractions in Rpt4-knockdown cells similar to Bag6-knockdown cells ( Fig. 3b and Supplementary Fig. S4 ). When these fractions were immunoprecipitated with Flag-Bag6, neither component of the p27 module was co-precipitated in control cells ( Fig. 3e ). In contrast, the p27-Rpt5 complex was co-precipitated in Rpt4-knockdown cells ( Fig. 3e ). We also confirmed the association of Bag6 with Rpt5 using an in vitro transcription–translation system ( Supplementary Fig. S5 ). These data suggest that Bag6 is associated with Rpt5 along with p27 and has a role in the recruitment of Rpt4 to this complex, which subsequently elicits the dissociation of Bag6 and assembly of the p27 module. In summary, Bag6 is not only involved in CP assembly as the most upstream component of the TRC pathway but also in the base assembly independent of the TRC pathway. The TRC pathway is not involved in the base assembly, as no RP assembly defect was observed in TRC40 knockdown. The precise mechanism by which the TRC pathway is involved in CP assembly remains unidentified. It is likely that some TA protein, together with UMP1 and propeptides of β-subunits, is responsible for efficient β-subunit assembly on α-rings ( Fig. 4 ). As ER association of the pre-CPs was compromised in TRC40 knockdown, such a TA protein on the ER membrane might serve as an acceptor for pre-CPs. Further studies are needed to identify this factor from ~400 predicted TA proteins [41] . 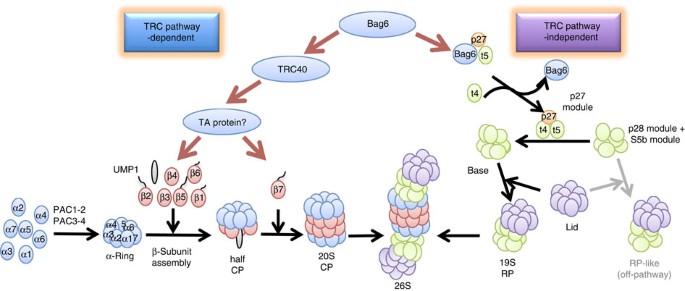Figure 4: A model of the roles of Bag6 and the TRC pathway in proteasome assembly. The TRC pathway, in which TA proteins chaperoned by Bag6 and TRC40 are delivered from ribosomes to the ER, is required for CP assembly by facilitating the incorporation of β-subunits on the α-ring or increasing the stabilities of CP assembly intermediates and subsequent dimerization of half-CPs. Bag6 also has a role in RP assembly, independent of the TRC pathway, by promoting formation of the p27-module. Figure 4: A model of the roles of Bag6 and the TRC pathway in proteasome assembly. The TRC pathway, in which TA proteins chaperoned by Bag6 and TRC40 are delivered from ribosomes to the ER, is required for CP assembly by facilitating the incorporation of β-subunits on the α-ring or increasing the stabilities of CP assembly intermediates and subsequent dimerization of half-CPs. Bag6 also has a role in RP assembly, independent of the TRC pathway, by promoting formation of the p27-module. Full size image Bag6 is a ribosome-associating chaperone that recognizes hydrophobic domains of nascent proteins and regulates protein triage, in which proteins undergo either productive folding and membrane targeting or ubiquitination and degradation [38] , [42] , [43] . Our findings add another layer of regulation for protein homoeostasis by Bag6 and the TRC pathway and have revealed that proteasome assembly is not an isolated system that is catalysed solely by dedicated chaperones but also requires general chaperones that preserve protein homoeostasis. Yeast genetics SGA screening was performed as described [25] . Yeast knockout strains were purchased from Open Biosystems (YSC1053). Yeast strain Y8025 and plasmid p4339 for SGA analysis were gifts from Dr. C. Boone (University of Toronto). Manual pin tools (Tokken) were used for SGA screening. See Supplementary Table S1 for genotypes of strains used. Biochemical analysis The cDNAs encoding Bag6 and TRC40 were isolated from HeLa cells by RT–PCR using total RNA. All constructs were confirmed by sequencing. Cells were lysed in a buffer containing 50 mM Tris-HCl (pH 7.5), 0.5% (v/v) NP-40, 1 mM dithiothreitol (DTT), 2 mM ATP and 5 mM MgCl 2 and clarified by centrifugation at 20,000 g for 15 min at 4 °C. For glycerol gradient analysis, clarified lysates were subjected to linear glycerol density gradient centrifugation with 4–24 or 8–32% glycerol in 25 mM Tris-HCl buffer (pH 7.5) containing 1 mM DTT and 2 mM ATP. After centrifugation at 83,000 g for 22 h, the gradient was separated into 32 fractions. The hydrolysis of the synthetic peptides, succinyl-Leu-Leu-Val-Tyr-7-amino-4-methylcoumarin (Suc-LLVY-MCA), was measured in 50 mM Tris-HCl (pH 8.0) containing 0.025% SDS. Antibodies against human TRC40 were raised in rat by immunizing recombinant His-TRC40 (residues 251–349). The anti-Bag6 polyclonal antibody was a gift from Dr. Kawahara (Tokyo Metropolitan University). The following antibodies were purchased and used at the indicated dilutions: ubiquitin (1:1,000; Dako), actin (1:1,000; Chemicon), GAPDH (1:1,000; Serotec), Derlin1 (1:1,000; MBL), Flag (1:1,000; Sigma), and β3 and β7 (1:500; BioMol). Other antibodies were described previously [21] , [31] , [32] , [36] . Densitometry analysis of the bands was performed using ImageQuant LAS4000 (GE Healthcare). For cell fractionation, cells were disrupted in a buffer containing 25 mM Tris-HCl (pH 7.5), 5 mM MgCl 2 , 250 mM sucrose and 1 mM DTT. The cell extracts were centrifuged at 8,000 g for 10 min. The resultant post-mitochondrial supernatant was further centrifuged at 100,000 g for 60 min, thus separating the supernatant cytosolic fraction and the sedimenting ER fraction. In vitro transcription–translation was performed using TnT T7 Quick systems (Promega). Knockdown experiments siRNA-mediated knockdown was performed as described previously [21] , [31] , [32] , [36] . The targeted sequences are as follows: TRC40, 5′-CAGACAACUUUCAUCUGCGUAUGCA-3′; Bag6, 5′-GCGCAUGUGCUGCAUUGCACAGAUA-3′; β7, 5′-GCAUGCGAGUGCUGUACUACC-3′; Rpt4, 5′-GAGAGAUUCAGAGAACGUUAAUGGA-3′. A negative control siRNA was purchased from Invitrogen. Cells were harvested 48 or 72 h after transfection of siRNA-targeting Rpt4 and β7 or TRC40 and Bag6, respectively. How to cite this article: Akahane, T. et al . Involvement of Bag6 and the TRC pathway in proteasome assembly. Nat. Commun. 4:2234 doi: 10.1038/ncomms3234 (2013)